Extrasynaptic vesicle recycling in mature hippocampal neurons Fast neuronal signalling relies on highly regulated vesicle fusion and recycling at specialized presynaptic terminals. Recently, examples of non-classical neurotransmission have also been reported, where fusion of vesicles can occur at sites remote from conventional synapses. This has potentially broad biological implications, but the underlying mechanisms are not well established. Here we show that a complete vesicle recycling pathway can occur at discrete axonal sites in mature hippocampal neurons and that extrasynaptic fusion is a robust feature of native tissue. We demonstrate that laterally mobile vesicle clusters trafficking between synaptic terminals become transiently stabilized by evoked action potentials and undergo complete but delayed Ca 2+ -dependent fusion along axons. This fusion is associated with dynamic actin accumulation and, subsequently, vesicles can be locally recycled, re-acidified and re-used. Immunofluorescence and ultrastructural work demonstrates that extrasynaptic fusion sites can have apposed postsynaptic specializations, suggesting that mobile vesicle recycling may underlie highly dynamic neuron–neuron communication. Most information transfer in the mature CNS relies on fast chemical transmission at synapses, ultrastructurally distinct neuron–neuron apposition points at which a presynaptic terminal harbouring a cluster of synaptic vesicles is located adjacent to a postsynaptic target. The specialized nature of these structures, which includes the complex arrays of proteins that regulate and mechanically facilitate the exocytic fusion of vesicles [1] , has led to the classical view that transmission occurs exclusively at such sites along the axon. In recent years, however, a new perspective on the independence of synaptic operation has emerged with novel examples of neuronal signalling that deviate from a simple point-to-point transmission model [2] , [3] . These include spillover, where transmitter released at one presynaptic terminal diffuses away from the synaptic cleft resulting in synaptic crosstalk and/or the activation of extrasynaptic receptors [4] , and ectopic transmission [2] , where vesicle fusion and transmitter release occur at sites away from anatomically defined presynaptic active zones [5] , [6] , [7] , [8] , [9] , [10] , [11] , [12] , [13] . In hippocampal neurons, a further departure from the classical model of synaptic transmission has come with the finding that recycling synaptic vesicles can be highly mobile, both in mature cultured neurons [14] , [15] , [16] , [17] , [18] and native tissue [17] , moving readily between synaptic release sites and participating in vesicle fusion at new synaptic hosts. As such, individual terminals essentially form part of a larger vesicle superpool [17] , [18] with important potential implications for axonal synapse–synapse interactions [17] , [19] , [20] . To date, attention has focused on the impact of mobile vesicles on recipient synaptic terminals [15] , [17] , but evidence also indicates that trafficking vesicles can be fusion-competent during transit, a property first reported in developing neurons [21] , [22] , [23] , [24] , [25] , [26] , [27] but since demonstrated in older cells [16] , [17] . Given the large number of trafficking vesicles moving along axons between established synapses [17] , axonal fusion in mature neurons could represent an important extra pathway for neuronal signalling. Here we have used a combination of exocytic and endocytic reporters of vesicle recycling, Ca 2+ imaging and correlative fluorescence and electron microscopy to characterize the dynamics and mechanisms underlying extrasynaptic vesicle fusion, both in native tissue and mature hippocampal neurons. We demonstrate that axonal segments of neurons in acute hippocampal slices can support fast fusion of mobile vesicles in response to action potentials. High-rate time-lapse imaging reveals the dynamics of this process: typically vesicles transiently stabilize before fusion and exocytose with fast release kinetics. Mobile vesicles can be recycled and reused outside synaptic terminals, and, using ultrastructural and fluorescence data, we show that these sites can be anatomically specialized and lie adjacent to postsynaptic targets. Our findings offer new insights into the presynaptic mechanics underlying an extra feature of information transmission in central neurons that deviates from the conventional model of point-to-point transmission and could signal dynamic aspects of neuronal function. Mobile vesicle fusion at axonal sites Recycling vesicles are highly mobile between synaptic terminals [14] , [15] , [16] , [17] , [18] as evidenced in time-lapse sequences ( Supplementary Fig. S1 ). Importantly, these trafficking vesicles can undergo fusion, both after integration into a synaptic host [15] , [17] or orphan synapse [16] , but also at times immediately following [16] or even during transit [17] . To test the relevance of this in native tissue, we characterized stimulus-evoked vesicle dynamics in acute hippocampal slices. Synaptic terminals in CA1 were loaded with FM1-43 (refs 28 , 29 ) by electrical stimulation (10 Hz 1,200 action potentials, AP) of Schaffer-collaterals [30] , [31] with field potential recordings confirming effective stimulation of the target CA1 region ( Fig. 1a ). After washing, fluorescence imaging revealed robust punctate staining ( Fig. 1b ) that could be rapidly destained with electrical stimulation ( n =18 slices from 5 animals), where the rate of fluorescence loss increased with stimulation frequency ( Fig. 1b,c ). Next, we looked for fluorescent trafficking puncta in time-lapse sequences [17] to test their stimulus-driven fusion-competence. Mobile packets were readily observed, both integrating into stable terminals ( Supplementary Fig. S2 ), but also trafficking linearly along unlabelled lengths of intersynaptic axon ( Fig. 1d ). We found that stimulation appeared to stabilize these packets and evoked reliable dye loss ( Fig. 1e,f ) with the rate and extent of destaining in mobile vesicles comparable to stable synaptic neighbours ( τ for stable: 14±5 s, τ for mobile: 15±7 s, n =15 and 11 from 3 slices from 2 animals, P =0.93, t -test, Fig. 1f ). 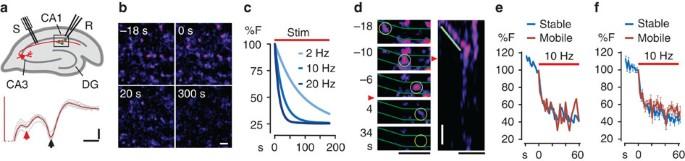Figure 1: Mobile vesicle fusion in acute slice. (a) Preparation used and electrical response to stimulation. FM-dye-loading of terminals in the stratum radiatum of CA1 is achieved by electrical stimulation (S) of Schaffer collaterals. Typical field excitatory postsynaptic potential recordings (grey lines) from target CA1 region (R) in the presence of AP5 are shown, with average trace in red. Vertical line on left shows the end of the stimulus artefact (stimulus: 1 ms). Red arrow is fibre volley. Black arrow is fEPSP. Vertical bar: 0.5 mV, Horizontal: 2 ms. (b) Sample images of fluorescent puncta and destaining at 10 Hz after 0 s. Scale bar, 2 μm. (c) Single exponential curve fits from average data showing stimulation-evoked dye loss at 2, 10 and 20 Hz (16, 47 and 19 synapses, respectively from 1 slice each from 2 animals). (d) Sample time-lapse images and kymograph showing FM-dye packet mobility and destaining. Red triangles indicate 10 Hz stimulation. Scale bar, 5 μm. Vertical bar, 10 s. (e) Destaining curve traces for packet from (d) (red) and seven stable neighbouring synapses (blue). (f) Summary destaining curves for mobile packets (n=11) and stable synaptic neighbours (n=15). Figure 1: Mobile vesicle fusion in acute slice. ( a ) Preparation used and electrical response to stimulation. FM-dye-loading of terminals in the stratum radiatum of CA1 is achieved by electrical stimulation (S) of Schaffer collaterals. Typical field excitatory postsynaptic potential recordings (grey lines) from target CA1 region (R) in the presence of AP5 are shown, with average trace in red. Vertical line on left shows the end of the stimulus artefact (stimulus: 1 ms). Red arrow is fibre volley. Black arrow is fEPSP. Vertical bar: 0.5 mV, Horizontal: 2 ms. ( b ) Sample images of fluorescent puncta and destaining at 10 Hz after 0 s. Scale bar, 2 μm. ( c ) Single exponential curve fits from average data showing stimulation-evoked dye loss at 2, 10 and 20 Hz (16, 47 and 19 synapses, respectively from 1 slice each from 2 animals). ( d ) Sample time-lapse images and kymograph showing FM-dye packet mobility and destaining. Red triangles indicate 10 Hz stimulation. Scale bar, 5 μm. Vertical bar, 10 s. ( e ) Destaining curve traces for packet from ( d ) (red) and seven stable neighbouring synapses (blue). ( f ) Summary destaining curves for mobile packets ( n =11) and stable synaptic neighbours ( n =15). Full size image Next, we turned to FM1-43-labelling in dissociated cultures, where we could characterize the processes that support extrasynaptic fusion in detail. We restricted our analysis to discrete packets that were mobile at the time of stimulation, remained at intersynaptic sites during the whole stimulation period and showed clear activity-evoked dye loss ( Fig. 2a ). To characterize the relationship between activity and vesicle movement, we generated kymographs for target packets ( Fig. 2b,c ) and measured the average rate of vesicle movement immediately preceding and following stimulus onset (40 Hz 1,200 AP). Again, we found a significant average reduction in mobility following the stimulus ( Fig. 2d ). Thus, overall, activity tends to result in stabilization of previously mobile packets at sites between conventional terminals. Nonetheless, it was clear that at the level of individual packets, more complex relationships between mobility and stimulation could sometimes be observed. We investigated this by categorizing movements for n =46 packets (12 coverslips from 7 culture preparations, or 12/7) across the range of experimental conditions used in this paper ( Fig. 2e ). After stimulation the majority of packets (61%) stabilized fully, but 28% continued to mobilize at a reduced rate and 11% moved at the same rate as before. To gain some insight into the incidence of mobile destaining, we next quantified the number of FM-dye-loss events occurring through mobile fusion in clearly defined axonal segments adjacent to stable synaptic boutons ( n =50 from 4/2, length: 3.5 μm). Our analysis revealed that along these segments, 29.5% of individual dye-loss events arose from mobile fusion. As such, this represents a substantial component of measured dye-loss events suggesting that this process has considerable potential relevance for signalling. 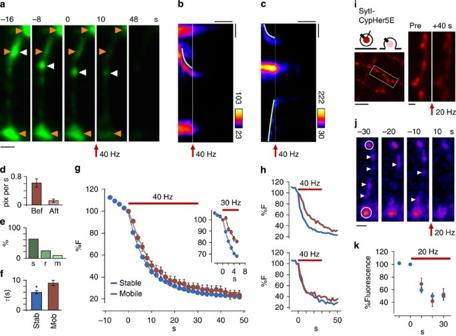Figure 2: Stimulation-evoked movement and fusion properties of mobile vesicles. (a) Time-lapse of axon of FM1-43-loaded neuron with fluorescently labelled stable terminals (orange arrowheads) and mobile packet (white arrowhead). Stimulation results in rapid dye loss. Scale bar, 1 μm. (b) Kymograph generated from a line scan along the axon of the same sequence from (a). Green line indicates profile of mobile packet. Scale bar, 1 μm. Horizontal: 20 s. (c) Second example kymograph with a stable synapse and two mobile packets (green lines). Scale bar, 1 μm. Horizontal: 20 s. (d) Histogram showing mean±s.e.m. mobility rates for trafficking packets before and after stimulation (pixels per sec before: 0.62±0.11, after: 0.12±0.04, pairedt-test,P<0.01,n=12 from 6/2). (e) Histogram showing % occurrence of three different categories of stimulation-evoked movement dynamics: s, stabilized; r, reduced trafficking rate; m, movement at pre-stimulation rate, forn=46 from 12/7. (f,g) Mean±s.e.m. FM1-43 destaining plots (g) for mobile vesicle packets (n=13 from 6/2) and stable terminals from adjacent regions (n=60). Lines are single exponential fits. inset: Mean±s.e.m. destaining plots using faster acquisition imaging reveals delayed dye loss in mobile packets versus stable synapses (n=6 from 2/1). (f) Mean±s.e.m.τfor single exponential curve fits from (g). (h) Sample destaining plots for two mobile packets (red lines), one moving at stimulation point (top) and one that spontaneously stabilized before stimulation (bottom). Neighbouring stable synapse traces are shown in blue. (i) SytI-CypHer5E (loading: 600 APs 10 Hz, left, Scale bar, 5 μm.) and stimulation-evoked quenching (right, Scale bar, 1 μm). (j) Time-lapse sequence of mobile SytI-CypHer5E packets along axons (white arrowheads) quenching with stimulation. Scale bar, 1 μm. (k) Mean±s.e.m. plots of stimulation-evoked fluorescence loss at stable terminals (n=24 from 3/2) and mobile packets (n=6 from 3/2). Figure 2: Stimulation-evoked movement and fusion properties of mobile vesicles. ( a ) Time-lapse of axon of FM1-43-loaded neuron with fluorescently labelled stable terminals (orange arrowheads) and mobile packet (white arrowhead). Stimulation results in rapid dye loss. Scale bar, 1 μm. ( b ) Kymograph generated from a line scan along the axon of the same sequence from ( a ). Green line indicates profile of mobile packet. Scale bar, 1 μm. Horizontal: 20 s. ( c ) Second example kymograph with a stable synapse and two mobile packets (green lines). Scale bar, 1 μm. Horizontal: 20 s. ( d ) Histogram showing mean±s.e.m. mobility rates for trafficking packets before and after stimulation (pixels per sec before: 0.62±0.11, after: 0.12±0.04, paired t -test, P <0.01, n =12 from 6/2). ( e ) Histogram showing % occurrence of three different categories of stimulation-evoked movement dynamics: s, stabilized; r, reduced trafficking rate; m, movement at pre-stimulation rate, for n =46 from 12/7. ( f , g ) Mean±s.e.m. FM1-43 destaining plots ( g ) for mobile vesicle packets ( n =13 from 6/2) and stable terminals from adjacent regions ( n =60). Lines are single exponential fits. inset: Mean±s.e.m. destaining plots using faster acquisition imaging reveals delayed dye loss in mobile packets versus stable synapses ( n =6 from 2/1). ( f ) Mean±s.e.m. τ for single exponential curve fits from ( g ). ( h ) Sample destaining plots for two mobile packets (red lines), one moving at stimulation point (top) and one that spontaneously stabilized before stimulation (bottom). Neighbouring stable synapse traces are shown in blue. ( i ) SytI-CypHer5E (loading: 600 APs 10 Hz, left, Scale bar, 5 μm.) and stimulation-evoked quenching (right, Scale bar, 1 μm). ( j ) Time-lapse sequence of mobile SytI-CypHer5E packets along axons (white arrowheads) quenching with stimulation. Scale bar, 1 μm. ( k ) Mean±s.e.m. plots of stimulation-evoked fluorescence loss at stable terminals ( n =24 from 3/2) and mobile packets ( n =6 from 3/2). Full size image Next, we examined mobile vesicle fusion kinetics. 40 Hz stimulation produced reliable destaining of mobile packets and stable terminals in the same field of view ( Fig. 2f,g ). This was also conserved in very mature neurons (DIV32, Supplementary Fig. S2 ). Overall, dye loss for mobile and stable puncta had a similar profile but the destaining time course was significantly slower for mobile packets ( τ for stable: 7±1 s, τ for mobile: 11±1 s, P <0.01, t -test, n =13 for each from 6/2, Fig. 2f ). We attributed this to delayed onset of dye loss, revealed in pairwise comparisons for the first 6 seconds after stimulation (stable versus mobile, 2 s: 0.80±0.03 and 0.91±0.03, P <0.01; 4 s: 0.63±0.04 and 0.76±0.03, P <0.01; 6 s: 0.54±0.04 and 0.68±0.04, P <0.01, t -tests) and supported by further experiments using faster acquisition imaging to visualize the initial destaining period ( Fig. 2g , stable versus mobile, 1 s: 0.90±0.01 and 1.02±0.01, P <0.01; 2 s: 0.81±0.01 and 0.92±0.01, P <0.03; 3 s: 0.75±0.01 and 0.89±0.02, P <0.01, t -tests, n =6 for each from 2/1). We reasoned this lag might correspond to a period required for vesicles to move to and/or become associated with an appropriate section of target membrane. To test this, we examined destaining profiles of mobile packets that had spontaneously stabilized several frames before stimulation. These packets underwent activity-evoked dye loss without delay when compared with destaining profiles from neighbouring control synapses (pairwise comparisons for first 3 points after stimulation, stable versus stabilized packet, 2 s: 0.84±0.02 and 0.86±0.01; 4 s: 0.71±0.06 and 0.73±0.03; 6 s: 0.61±0.06 and 0.58±0.04, P >0.25, paired t -test for all, n =4 for each from 3/2 ( Fig. 2h ). Thus, steps required to change mobile vesicles into fusion-competent vesicles could be sufficient to account for a delayed onset to exocytosis. To confirm our findings, we next tested an alternative vesicle reporter, SytI-CypHer5E, based on a fluorescent-conjugated antibody targeted to the luminal domain of the vesicle protein synaptotagmin [32] . CypHer5E is pH-sensitive, fluorescing strongly in the acidic vesicle lumen, but quenched when the fluorophore is exposed to neutral extracellular pH ( Fig. 2i ). Thus it provides a sensitive readout of intact, recently recycled, acidified vesicles. As expected, SytI-CypHer5E puncta underwent stimulation-evoked fluorescence quenching as vesicles fused with the membrane ( Fig. 2i ). Moreover, time-lapse imaging sequences revealed laterally mobile packets of vesicles that underwent stimulation-evoked fluorescence loss ( τ for stable: 7±2 s, τ for mobile: 12±2 s, n =24 and n =6 from 3/2, P =0.08, t -test, Fig. 2j,k ). These results, using a different vesicle probe, support our FM-dye findings. The experiments described so far have relied on recycling vesicle probes that label functional vesicle pools. Next, we considered whether axonal sites supporting mobile fusion might, in fact, be presynaptically silent synapses containing non-recycling vesicles that are functionally engaged by the arrival of recycling ones. We performed dual-imaging time-lapse experiments using FM1-43 and synaptophysinI-mCherry (SypI-mCherry) ( Fig. 3a ), a non-selective marker of vesicles, to examine the specific dependency of a site where mobile fusion takes place on the prior presence of mCherry fluorescence. Although, as expected, SypI-mCherry and FM-fluorescence were co-localized in trafficking packets, mobile vesicle fusion events could readily occur at sites that were previously SypI-mCherry-negative ( Fig. 3a,b ). Thus, target fusion sites without pre-existing pools of vesicles can support mobile exocytosis. 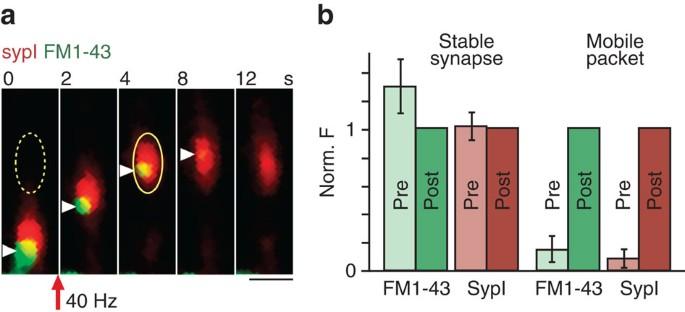Figure 3: Fusion occurs at previously vesicle-free sites along axons. (a) Example time-lapse imaging experiment of FM1-43 fluorescence in SypI-mCherry-expressing neuron, showing that mobile fusion (white arrowhead) can take place at novel sites not already populated with vesicles. Yellow ovals indicate axonal site of destaining. Scale bar, 1 μm. (b) Quantification of experiments in (a). Histograms show FM1-43 (green) and SypI-mCherry (red) fluorescence at fusion sites for mobile packets and neighbouring stable terminals (n=4 from 3/3). 'Pre' corresponds to the fluorescence for each region at the time point where mCherry signal is at its lowest for the mobile packet. 'Post' represents the time point after the packet has stabilized at the destaining site. All values are normalized to post-fluorescence values for each condition. The histogram shows that before the arrival of the mobile packet at the axonal site, FM1-43 and mCherry fluorescence are close to background levels. Values are mean±s.e.m. Figure 3: Fusion occurs at previously vesicle-free sites along axons. ( a ) Example time-lapse imaging experiment of FM1-43 fluorescence in SypI-mCherry-expressing neuron, showing that mobile fusion (white arrowhead) can take place at novel sites not already populated with vesicles. Yellow ovals indicate axonal site of destaining. Scale bar, 1 μm. ( b ) Quantification of experiments in ( a ). Histograms show FM1-43 (green) and SypI-mCherry (red) fluorescence at fusion sites for mobile packets and neighbouring stable terminals ( n =4 from 3/3). 'Pre' corresponds to the fluorescence for each region at the time point where mCherry signal is at its lowest for the mobile packet. 'Post' represents the time point after the packet has stabilized at the destaining site. All values are normalized to post-fluorescence values for each condition. The histogram shows that before the arrival of the mobile packet at the axonal site, FM1-43 and mCherry fluorescence are close to background levels. Values are mean±s.e.m. Full size image Axonal fusion sites can support endocytosis Next, we tested whether extrasynaptic fusion sites can support endocytosis and local vesicle reuse. SytI-CypHer5E is an informative tool to address this question, because it reports both the exocytic phase of vesicle turnover, but also the endocytic leg as a recovery in fluorescence signal when retrieved vesicles are re-acidified and CypHer5E fluorescence becomes unquenched ( Fig. 4a,b ). Although the high sensitivity of CypHer5E to photobleaching precluded a detailed analysis of endocytic properties of mobile vesicles, fluorescence recovery after stimulation was seen ( Fig. 4b,c ). Thus, a mobile vesicle packet can undergo fusion, endocytosis and re-acidification at an axonal site distinct from a conventional terminal, and then become mobilized again. Next, we examined this with SypHyx2, that reports vesicle exocytosis with a rise in fluorescence and quenches when recycling vesicles become re-acidified after endocytosis [33] ( Fig. 4d,e ). We found that stimulation could bring about an initial increase in fluorescence signal in these packets ( Fig. 4e ) reflecting vesicle fusion and consistent with our FM-dye data. Moreover, confirming our SytI-CypHer5E findings, we also recorded a subsequent signal reduction, corresponding to endocytosis and re-acidification ( Fig. 4d,e ). Overall, the average time course of endocytosis from all mobile packets was comparable to stable control synapses ( τ for stable: 46 s, τ for mobile: 49 s, n =40 and n =7 from 3/3, Fig. 4d ) suggesting that the two groups shared similar underlying endocytic mechanisms. Taken together, our findings show that mobile vesicles can undergo a complete recycling pathway typically correlated with a stabilization of mobile vesicles ( Fig. 4e ). Finally, we examined whether packets could undergo multiple rounds of fusion. Neurons were subjected to a paired stimulation protocol evoking a reliable double rise in fluorescence in stable synapses and mobile packets ( n =3 from 3/2, Fig. 4f,g ), supporting the idea that mobile vesicles could engage in repeated vesicle recycling events. 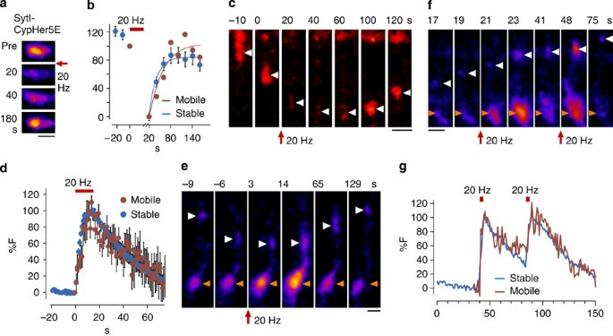Figure 4: Axonal fusion sites support vesicle endocytosis, re-acidification and reuse. (a,b) Image sequence and plot of CypHer5E fluorescence showing recovery of signal after stimulation (400 APs, 20 Hz) at a stable synaptic terminal (a) and mean±s.e.m. fluorescence plot (b) reflecting the endocytosis and re-acidification of vesicles (n=13 stable synapses from 1 coverslip). Scale bar, 1 μm. Note the change in timescale along x axis after stimulation. Red points are associated with recovery of the mobile packet from (c) (n=1 from 1 coverslip). (c) Time-lapse of a SytI-CypHer5E-labelled mobile vesicle packet (white arrowheads) showing mobility, stabilization, activity-evoked fusion, re-acidification and remobilization. Scale bar, 1 μm. (d,e) Endocytosis in mobile packets examined using SypHyx2. (d) Summary plot of responses in mobile packets (n=7 from 3/3, red) and stable terminals (n=40, blue). Points are mean±s.e.m. (e) Sample time-lapse sequence showing mobile packet (white arrowhead) and neighbouring stable terminal (orange arrowhead) exhibiting a fluorescence rise on stimulation (0–15 s). Scale bar, 1 μm. (f) Sample time-lapse frames showing a mobile packet (white arrowhead) as well as a stable synapse (orange arrowhead) undergoing multiple fusion events with two rounds of 20 Hz stimulation. Scale bar, 1 μm. (g) Mean plots showing responses to dual stimulation protocol for mobile packets (n=3, from 3/2, red) and their neighbouring stable terminals (n=3, blue). For clarity, s.e.m. error bars are not shown. Figure 4: Axonal fusion sites support vesicle endocytosis, re-acidification and reuse. ( a , b ) Image sequence and plot of CypHer5E fluorescence showing recovery of signal after stimulation (400 APs, 20 Hz) at a stable synaptic terminal ( a ) and mean±s.e.m. fluorescence plot ( b ) reflecting the endocytosis and re-acidification of vesicles ( n =13 stable synapses from 1 coverslip). Scale bar, 1 μm. Note the change in timescale along x axis after stimulation. Red points are associated with recovery of the mobile packet from (c) ( n =1 from 1 coverslip). ( c ) Time-lapse of a SytI-CypHer5E-labelled mobile vesicle packet (white arrowheads) showing mobility, stabilization, activity-evoked fusion, re-acidification and remobilization. Scale bar, 1 μm. ( d , e ) Endocytosis in mobile packets examined using SypHyx2. ( d ) Summary plot of responses in mobile packets ( n =7 from 3/3, red) and stable terminals ( n =40, blue). Points are mean±s.e.m. ( e ) Sample time-lapse sequence showing mobile packet (white arrowhead) and neighbouring stable terminal (orange arrowhead) exhibiting a fluorescence rise on stimulation (0–15 s). Scale bar, 1 μm. ( f ) Sample time-lapse frames showing a mobile packet (white arrowhead) as well as a stable synapse (orange arrowhead) undergoing multiple fusion events with two rounds of 20 Hz stimulation. Scale bar, 1 μm. ( g ) Mean plots showing responses to dual stimulation protocol for mobile packets ( n =3, from 3/2, red) and their neighbouring stable terminals ( n =3, blue). For clarity, s.e.m. error bars are not shown. Full size image Dynamic recruitment of actin to sites of axonal fusion Actin is an important and highly dynamic cytoskeletal element that is concentrated at synapses [34] , [35] ( Fig. 5a ), and implicated as a synaptic scaffolding element supporting vesicle turnover [35] , in synaptic remodelling [34] and in lateral vesicle trafficking [15] , [18] . We reasoned that actin remodelling might accompany or even facilitate the vesicle movement along axons, and support recycling events. To test this, we labelled GFP-actin-expressing neurons with the vesicle marker SytI-Oyster550 ( Fig. 5a ) and monitored dynamic movements with dual-colour time-lapse imaging. Vesicle movements to new sites along the axon were associated with directed recruitment of actin ( Fig. 5b ) but aggregation followed, rather than preceded, the mobilization of vesicle packets ( Fig. 5b,c ). Moreover, fusion-competence of mobile vesicles did not appear to be critically dependent on the presence of actin because effective activity-evoked dye loss could occur before significant actin condensation ( Fig. 5d,e ). 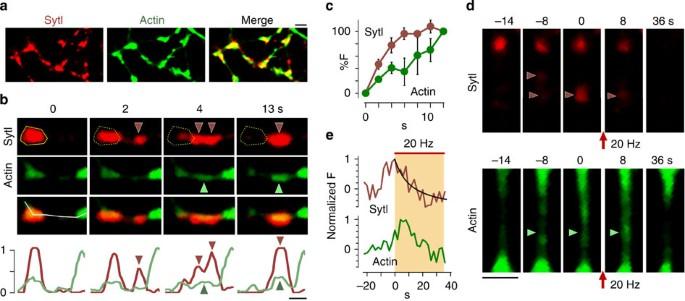Figure 5: Recruitment of actin to mobile vesicle packets. (a) Images showing co-localization of SytI-Oyster550 (red) and GFP-actin (green) in actin-transfected neurons. Scale bar, 1 μm. (b) Sample time-lapse images showing movement of vesicle packet (red arrowheads) followed by aggregation of actin to the same site (green arrowheads) and corresponding fluorescence profiles. Scale bar, 1 μm. (c) Summary mean±s.e.m. data plots for vesicle movement events fromn=5 packets (red) and actin (green) from 2 coverslips from culture preparations. Data show average fluorescence in the region of interest into which the packet moved. Data is normalized to peak in actin fluorescence illustrating the kinetics of fluorescence turnover. (d) (Left) sample time-lapse images showing movement of a SytI-Oyster550-labelled vesicle packet (red arrowhead) to new site before undergoing activity-evoked vesicle fusion with 20 Hz stimulation, and corresponding images for GFP-actin (green). Scale bar, 1 μm. (e) Plots for SytI-Oyster and actin from (d). Activity-evoked dye loss is shown with single exponential fit. Figure 5: Recruitment of actin to mobile vesicle packets. ( a ) Images showing co-localization of SytI-Oyster550 (red) and GFP-actin (green) in actin-transfected neurons. Scale bar, 1 μm. ( b ) Sample time-lapse images showing movement of vesicle packet (red arrowheads) followed by aggregation of actin to the same site (green arrowheads) and corresponding fluorescence profiles. Scale bar, 1 μm. ( c ) Summary mean±s.e.m. data plots for vesicle movement events from n =5 packets (red) and actin (green) from 2 coverslips from culture preparations. Data show average fluorescence in the region of interest into which the packet moved. Data is normalized to peak in actin fluorescence illustrating the kinetics of fluorescence turnover. ( d ) (Left) sample time-lapse images showing movement of a SytI-Oyster550-labelled vesicle packet (red arrowhead) to new site before undergoing activity-evoked vesicle fusion with 20 Hz stimulation, and corresponding images for GFP-actin (green). Scale bar, 1 μm. ( e ) Plots for SytI-Oyster and actin from ( d ). Activity-evoked dye loss is shown with single exponential fit. Full size image Postsynaptic targets and ultrastructure Mobile fusion will have particular relevance, if recycling can occur at sites apposed to postsynaptic targets. To examine this, we combined FM-dye destaining with co-labelling for postsynaptic markers. In our cultures, stable puncta appeared to be co-apposed to postsynaptic targets in nearly all cases (glutamate receptor 1 (GluR1): 90±3%, n =920 synapses, 4/1; PSD-95: 91±3%, n =999 synapses, 3/1; GABA (γ-aminobutyric acid)-A-R: 35±7%, n =752 synapses, 5/2). Mobile fusion events onto target structures were readily observed (GluR1 or GluR2, n =20 examples from 6/2; GABA-A-R, n =5 from 3/2) (see Fig. 6a-d ). Notably, a variety of dynamic relationships were apparent between mobile packets and their targets. For example, postsynaptic markers could be presynaptically unapposed before the arrival of a packet ( Fig. 6b ) or, alternatively, host other transient presynaptic traffic ( Fig. 6c ). Also, evoked dye loss could be delayed until a mobile packet trafficked to a postsynaptic site ( Fig. 6c , middle). Although mobility of synaptic vesicles was high, coordinated lateral movement of postsynaptic label was not seen ( Fig. 6e,f ). Consistent with previous work [16] , we also observed some mobile packets that destained at sites that did not seem to be intimately associated with specific postsynaptic markers although these were more confined to isolated processes in sparse regions of the culture. 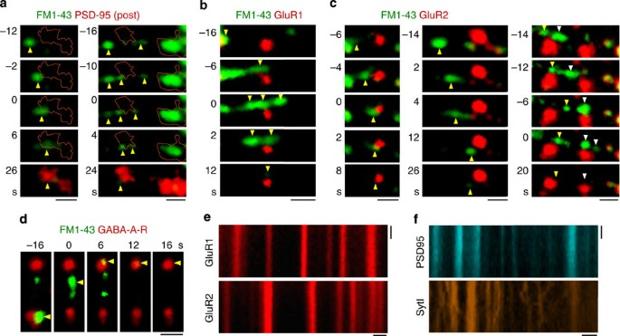Figure 6: Postsynaptic targets for mobile fusion. (a) Sample panels from time-lapse sequences showing movement and destaining (40 Hz after 0 s) of mobile FM1-43-labelled packets (arrowheads). Bottom panels show post-fix anti-PSD-95 with Alexa 568 immunostaining. Scale bars, 1 μm. (b,c) Sample panels from dual-imaging time-lapse sequences showing movement and destaining (40 Hz after 0 s) of mobile FM1-43-labelled packets (arrowheads) and live antibody labelling for GluR1 or GluR2. Mobile packets move to sites adjacent to GluR targets and destain. Scale bars, 1 μm. (d) Sample panels from dual-imaging time-lapse sequence showing movement and destaining (40 Hz after 0 s) of mobile FM1-43-labelled packets (arrowheads) and live antibody labelling for GABA-A receptor. Scale bar, 1 μm. (e) Sample kymographs showing the lack of lateral movement of GluR. Scale bar, 1 μm. Vertical time bar, 10 s. (f) Sample kymograph showing no evidence of lateral movement of ECFP-PSD-95 whereas the trafficking of vesicles labelled with SytI-Oyster550 along the apposed process is clearly evident. Scale bar, 2 μm. Vertical time bar, 10 s. Figure 6: Postsynaptic targets for mobile fusion. ( a ) Sample panels from time-lapse sequences showing movement and destaining (40 Hz after 0 s) of mobile FM1-43-labelled packets (arrowheads). Bottom panels show post-fix anti-PSD-95 with Alexa 568 immunostaining. Scale bars, 1 μm. ( b , c ) Sample panels from dual-imaging time-lapse sequences showing movement and destaining (40 Hz after 0 s) of mobile FM1-43-labelled packets (arrowheads) and live antibody labelling for GluR1 or GluR2. Mobile packets move to sites adjacent to GluR targets and destain. Scale bars, 1 μm. ( d ) Sample panels from dual-imaging time-lapse sequence showing movement and destaining (40 Hz after 0 s) of mobile FM1-43-labelled packets (arrowheads) and live antibody labelling for GABA-A receptor. Scale bar, 1 μm. ( e ) Sample kymographs showing the lack of lateral movement of GluR. Scale bar, 1 μm. Vertical time bar, 10 s. ( f ) Sample kymograph showing no evidence of lateral movement of ECFP-PSD-95 whereas the trafficking of vesicles labelled with SytI-Oyster550 along the apposed process is clearly evident. Scale bar, 2 μm. Vertical time bar, 10 s. Full size image To gain further insight into the structural organization of mobile fusion sites, we next subjected fusion-competent trafficking vesicles to ultrastructural analysis. During imaging, FM-dye-labelled synapses were partially destained via field stimulation (120 AP, 30 Hz, Fig. 7a,b ), then immediately fixed and photoconverted so that FM-dye-containing vesicles become electron-dense ( Fig. 7a ) [36] , [37] , [38] . Imaging revealed fusion-competent mobile packets ( n =4 from 1/1, Fig. 7c ) that we could target in the electron microscope using correlative methods outlined previously ( Fig. 7d-f ) [15] , [39] . At the ultrastructural level, all target packets consisted of a loosely arranged cluster of photoconverted and non-photoconverted vesicles, corresponding to recycling and non-recycling vesicles, respectively ( Fig. 7g–i , Supplementary Fig. S3 ). The mean percentage of recycling vesicles relative to total vesicles was 34±9% ( n =4). Notably, all analysed packets contained docked vesicles (mean: 1.5±0.5, n =4) and were along an axonal section that was intimately apposed to a postsynaptic structure ( Fig. 7g ), showing that these were not orphan sites. Thus, mobile vesicle clusters can fuse at regions of the axon that have many structural features found in conventional terminals, and would therefore be relevant for neuron–neuron signalling. 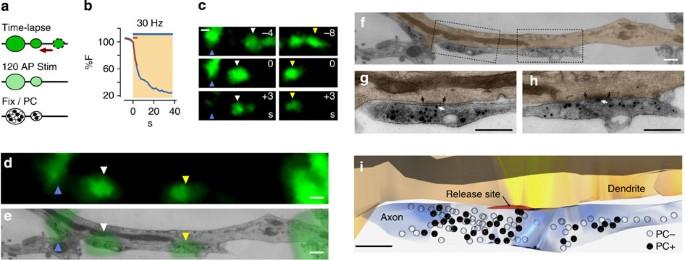Figure 7: Ultrastructure of axonal fusion sites. (a) Schematic of experiment. Neurons were loaded with FM1-43FX and imaged during stimulation (120 AP, 30 Hz) after which they were fixed, photoconverted (PC) and prepared for electron microscopy. (b) Mean destaining traces showing that before fixing, dye loss for 120 AP stimulation protocol (red) was equivalent to a sister culture where stimulation was maintained (blue). (c) Left, sample time-lapse frames from a target region showing a mobile packet (white arrowhead) moving to new site and undergoing stimulation-evoked dye loss in a typically delayed manner compared with the adjacent stable synapse (blue arrowhead). Right, example of mobile packet (yellow arrowhead) merging with another small packet and undergoing destaining. Scale bar, 0.5 μm. (d) Fluorescence image showing target site from (c) with arrowheads marking the same structures. (e) Electron micrograph of target region from (d) with fluorescence overlay illustrating correlative approach. (f) Electron micrograph of same region from (e) with dendrite marked in brown and mobile release sites indicated with dashed rectangles. Scale bars for (d–f): 0.5 μm. (g) High-magnification electron micrograph of left target region (dashed rectangle) from (f). (h) High-magnification electron micrograph of right target region (dashed rectangle) from (f). Both (g) and (h) show vesicles with dark lumen corresponding to recycling vesicles, docked vesicles (white arrowheads) and specialized postsynaptic structures (black arrows). Scale bars for (g) and (h): 0.5 μm. (i) Reconstruction for release site in (g). Scale bar, 0.25 μm. Figure 7: Ultrastructure of axonal fusion sites. ( a ) Schematic of experiment. Neurons were loaded with FM1-43FX and imaged during stimulation (120 AP, 30 Hz) after which they were fixed, photoconverted (PC) and prepared for electron microscopy. ( b ) Mean destaining traces showing that before fixing, dye loss for 120 AP stimulation protocol (red) was equivalent to a sister culture where stimulation was maintained (blue). ( c ) Left, sample time-lapse frames from a target region showing a mobile packet (white arrowhead) moving to new site and undergoing stimulation-evoked dye loss in a typically delayed manner compared with the adjacent stable synapse (blue arrowhead). Right, example of mobile packet (yellow arrowhead) merging with another small packet and undergoing destaining. Scale bar, 0.5 μm. ( d ) Fluorescence image showing target site from ( c ) with arrowheads marking the same structures. ( e ) Electron micrograph of target region from ( d ) with fluorescence overlay illustrating correlative approach. ( f ) Electron micrograph of same region from ( e ) with dendrite marked in brown and mobile release sites indicated with dashed rectangles. Scale bars for ( d – f ): 0.5 μm. ( g ) High-magnification electron micrograph of left target region (dashed rectangle) from ( f ). ( h ) High-magnification electron micrograph of right target region (dashed rectangle) from ( f ). Both ( g ) and ( h ) show vesicles with dark lumen corresponding to recycling vesicles, docked vesicles (white arrowheads) and specialized postsynaptic structures (black arrows). Scale bars for ( g ) and ( h ): 0.5 μm. ( i ) Reconstruction for release site in ( g ). Scale bar, 0.25 μm. Full size image Action potential dependent Ca 2+ entry at axonal sites Exocytosis requires a rapid increase in local [Ca 2+ ] (ref. 40 ). However, Ca 2+ increases along the axon are known to be smaller and slower than in synaptic terminals [41] , [42] , raising questions about how axonal sites could support vesicle fusion. To address this, we first confirmed the dependency of mobile vesicle fusion on the presence of extracellular Ca 2+ by quantifying the stimulation-evoked dye loss in mobile vesicle packets (% dye loss corrected for photobleaching after 600 APs, 2.5 mM,: 45±8%, n =6 from 2/1; 0 mM: 4±3%, n =10 from 2/1, t -test, P <0.01). Next, we performed calcium imaging experiments to provide information on the kinetics of Ca 2+ entry along axonal segments between conventional terminals. We expressed the fusion construct SypI-mCherry to label presynaptic terminals and filled transfected neurons with the calcium indicator OGB-1 (200 μM) via whole-cell patch clamp ( Fig. 8a ). We then targeted mCherry-positive synapses and their flanking axon and imaged OGB-1 fluorescence with line scans during single-action potentials evoked via the patch-pipette. As expected [41] , we recorded reliable and rapid rises in Ca 2+ at synaptic terminals, and also established that these signals were not saturated ( Supplementary Fig. S4 ). At sites along the flanking axon, smaller and slower Ca 2+ changes could be observed, although these were still significantly above baseline ( Fig. 8b ). Importantly, though, the distinction between Ca 2+ dynamics at synaptic and non-synaptic regions was not always apparent. In 57% of axonal segments ( n =7 from 7/2 with an average length of 4.0±0.2 μm), we also observed 'hotspots' of fast and substantial Ca 2+ increases that were not correlated with stable SypI-mCherry positive puncta ( Fig. 8c–e ). At these sites, the peak Ca 2+ rise was the same as at synaptic sites (1.02±0.15, P >0.05, Δ F / F 0 normalized to neighbouring synaptic region, t -test, n =4 from 4/2, Fig. 8d,f ), whereas intermediate axonal sections were significantly different (0.17±0.07, P <0.01, t -test). Moreover, synapses and 'hotspots' had a similar fast rise time, and this was different to responses at intermediate axonal sites ( Fig. 8d,f ; synapse 11.32±1.76 ms; 'hotspot' 12.67±1.82 ms; axon 28.32±2.99 ms, ANOVA (analysis of variance) F(2,9)=17.38, P <0.001, Tukey's test S versus H, S versus A, H versus A; P >0.05, P <0.01, P <0.01, n =4). On repeated stimulation, 'hotspots' exhibited consistent responses suggesting that they were reliable loci for activity-dependent Ca 2+ entry ( Fig. 8e ). We also performed experiments using the lower affinity calcium indicator, Fluo-5F on SypI-mCherry-transfected neurons. We identified hotspots in three out of six axonal segments (from 6/1) and, again, found peak, rise times and decay times, equivalent to those for stable synapses ( Supplementary Fig. S5 ). 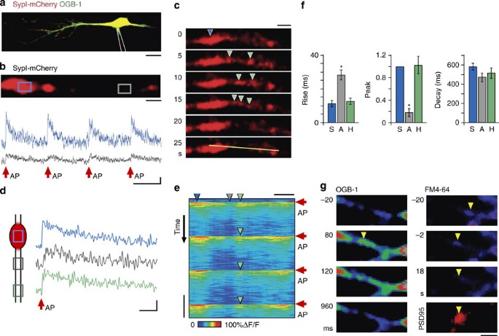Figure 8: Action potential dependent Ca2+entry at axonal sites. (a) Image overlay showing a SypI-mCherry-expressing neuron (red) filled with OGB-1 (green). The pipette is indicated with white lines. Scale bar, 10 μm. (b) Four single-action potential-evoked Ca2+responses at a synapse (blue box) and the flanking axonal region (grey box) marked in fluorescence image (top). Scale bar, 1 μm. Timescale bar 1 s. Vertical scale bar: 20% ΔF/F. (c) Time-lapse sequence showing movement of SypI-mCherry packets (green arrowheads) along axonal region next to stable synapse (blue arrowhead). Scale bar, 1 μm. (d) Sample Ca2+response traces from (c). Blue trace is stable synapse, grey trace is axonal region and green trace is Ca2+'hotspot' (e). Timescale bar 100 ms. Vertical scale bar: 50% ΔF/F. (e) Line scan (yellow line inc) showing Ca2+responses to four single-action potentials. Blue arrowhead, stable synapse; grey arrowhead, axonal region; green arrowheads, Ca2+'hotspot'. Scale bar, 1 μm. Timescale bar, 1 s. (f) Histograms showing mean±s.e.m. for 3 parameters of Ca2+response (n=4 from 4/2, with each sample averaged from 4 action potential-evoked responses) for synapse (S), axon (A) and 'hotspot' (H). For clarity, normalized ΔF/F0values are shown in histogram. Raw ΔF/F0were synapse, 0.58±0.13; hotspot: 0.57±0.16; and axon: 0.09±0.05 (n=4, each averaged from 4 responses). (g) Sample of experiment monitoring action potential-evoked Ca2+responses and FM-64 destaining sequentially. Time-lapse frames on left show rise in OGB-1-AM fluorescence evoked by single-action potential. Yellow arrowhead indicates 'hotspot'. (right) Time-lapse frames immediately following Ca2+imaging showing movement and dye loss of mobile packet (arrowhead) at the same site with 40 Hz stimulation. Bottom right panel shows post-fix immunolabelling of anti-PSD-95 with Alexa 568 indicating apposition to postsynaptic target at destaining site. Scale bar 1 μm. Figure 8: Action potential dependent Ca 2+ entry at axonal sites. ( a ) Image overlay showing a SypI-mCherry-expressing neuron (red) filled with OGB-1 (green). The pipette is indicated with white lines. Scale bar, 10 μm. ( b ) Four single-action potential-evoked Ca 2+ responses at a synapse (blue box) and the flanking axonal region (grey box) marked in fluorescence image (top). Scale bar, 1 μm. Timescale bar 1 s. Vertical scale bar: 20% Δ F / F . ( c ) Time-lapse sequence showing movement of SypI-mCherry packets (green arrowheads) along axonal region next to stable synapse (blue arrowhead). Scale bar, 1 μm. ( d ) Sample Ca 2+ response traces from ( c ). Blue trace is stable synapse, grey trace is axonal region and green trace is Ca 2+ 'hotspot' ( e ). Timescale bar 100 ms. Vertical scale bar: 50% Δ F / F . ( e ) Line scan (yellow line in c ) showing Ca 2+ responses to four single-action potentials. Blue arrowhead, stable synapse; grey arrowhead, axonal region; green arrowheads, Ca 2+ 'hotspot'. Scale bar, 1 μm. Timescale bar, 1 s. ( f ) Histograms showing mean±s.e.m. for 3 parameters of Ca 2+ response ( n =4 from 4/2, with each sample averaged from 4 action potential-evoked responses) for synapse (S), axon (A) and 'hotspot' (H). For clarity, normalized Δ F / F 0 values are shown in histogram. Raw Δ F / F 0 were synapse, 0.58±0.13; hotspot: 0.57±0.16; and axon: 0.09±0.05 ( n =4, each averaged from 4 responses). ( g ) Sample of experiment monitoring action potential-evoked Ca 2+ responses and FM-64 destaining sequentially. Time-lapse frames on left show rise in OGB-1-AM fluorescence evoked by single-action potential. Yellow arrowhead indicates 'hotspot'. (right) Time-lapse frames immediately following Ca 2+ imaging showing movement and dye loss of mobile packet (arrowhead) at the same site with 40 Hz stimulation. Bottom right panel shows post-fix immunolabelling of anti-PSD-95 with Alexa 568 indicating apposition to postsynaptic target at destaining site. Scale bar 1 μm. Full size image Taken together, our findings suggest that activity-evoked Ca 2+ rises occur throughout the axon but specific sites along axonal segments can support the fast action potential-evoked Ca 2+ rises necessary for axonal vesicle fusion. To test this directly, we carried out experiments using the membrane permeable form of OGB-1 (OGB-1-AM) in which we monitored stimulation-evoked Ca 2+ dynamics along axons followed immediately by time-lapse-imaging of FM-dye-destaining at the same sites. We found that fusion-competent mobile packets ( n =5 from 3/2) destained at sites where a discrete and substantial localized rise in Ca 2+ also occurred, equivalent to those we characterized above. For two of these, we also carried out post-fix immunolabelling and revealed a PSD-95-positive signal, consistent with the idea that fusion-sites can be relevant to postsynaptic signalling ( Fig. 8g ). Importantly, examples of mobile packets that did not undergo dye loss ( n =5 from 3/2, mean dye loss for 5 frames after stimulation: 3±1 versus 26±6% for fusion-competent packets, P <0.05, t -test) were present at sites with a much smaller rise in Ca 2+ signal than for fusion-competent packets (raw Δ F / F 0 : 0.09±0.02 versus 0.40±0.06, n =5, P <0.01, t -test). Thus, the capability of mobile vesicle clusters to undergo destaining and a stimulus-evoked rise in Ca 2+ at fusion sites are directly related. Using hippocampal neurons from mature cultures and acute slice, we have characterized key dynamic features of vesicle turnover along axons. Mobile fusion, in which discrete axonal regions behave as transiently active signalling sites contingent on the presence of trafficking vesicles, is an important departure from the conventional model of point-to-point neurotransmission. Our findings are compatible with studies in other systems that have detailed processes of ectopic or extrasynaptic transmission [5] , [6] , [7] , [8] , [9] , [10] , [11] , [12] , [13] . In particular, these examples have provided valuable information on how non-synaptic vesicle fusion can have a functional role in signalling to other neuronal [5] or non-neuronal targets [7] , [9] , [11] . Nonetheless, insights into presynaptic processes that facilitate Ca 2+ -dependent release of vesicles at axonal sites away from conventional synaptic terminals have not been directly addressed. Our findings here show that axonally derived signalling is a consequence of the fusion of trafficking vesicles arising from the laterally mobile vesicle pool [14] , [15] , [16] , [17] , [18] , [24] , [43] , [44] . These vesicles are typically stabilized by action potentials and subsequently undergo fast exocytosis. Notably, the onset of fusion is delayed, consistent with a period in which vesicles might be interacting with target proteins at axonal sites before exocytosis can occur; in support of this, we show that mobile vesicle packets that had spontaneously stabilized just before stimulation could undergo exocytosis immediately. Also, we noted examples of packets that delayed stimulus-evoked dye loss until they reached a GluR-apposed target region; we speculate that perhaps these packets do not immediately access molecular machinery required to support fusion. Using endocytic reporters, we demonstrate that vesicles involved in mobile fusion can be re-acidified and re-mobilized and subsequently undergo further fusion events. Thus, mobile vesicles, like those at conventional terminals [45] , can be locally recycled to support ongoing signalling demands. A confounding feature of regulated axonal fusion/recycling is that it runs against the established idea that Ca 2+ -dependent vesicle turnover is completely reliant on stably arranged, highly specialized presynaptic terminals. Our findings offer some insight into this. We demonstrate that sites along the axon that are not associated with stable synaptic terminals can support reliable action-potential-dependent rises in intracellular Ca 2+ with kinetics comparable to those at conventional terminals. Such sites were readily distinguishable from typical axonal segments where stimulus-driven Ca 2+ changes were smaller and slower, as reported previously [41] , [42] and which presumably arise in large part from the lateral spread of Ca 2+ from nearby terminals. Ca 2+ 'hotspots' would appear to provide the necessary large local rise in Ca 2+ to support mobile fusion of trafficking vesicles. Consistent with our findings, a recent work in corpus callosal neurons has demonstrated axonal release involving highly localized calcium microdomain signalling [7] . Another issue is how is the necessary vesicle recycling machinery might be made available for turnover of vesicles in axonal regions? A previous work has demonstrated that packets of laterally mobile vesicles can label immunopositive for synaptic proteins [16] , suggesting that some critical recycling machinery might already be present near fusion sites for local recruitment to trafficking vesicles; for example, the target soluble NSF attachment proteins receptors are known to be homogeneously distributed along axonal membranes [46] . However, our findings are not consistent with the idea that axonal release sites are small presynaptically silent synapses that become functionalized by the arrival of recycling vesicles because fusion events can readily occur at sites without a pre-existing vesicle pool. Alternatively, some synaptic components could themselves traffic to axonal sites to support mobile release consistent with work showing that many synapse-related elements are highly laterally mobile [47] , [48] , [49] , [50] , [51] , [52] , [53] . We demonstrate that actin is dynamically recruited to mobile vesicle packets. Interestingly, this recruitment occurs with some delay, suggesting that actin might not be critical for mobile fusion per se but acts in a supporting function, similar to its proposed role in stable terminals [35] . The fact that we observe mobile recycling in mature cultured neurons and native tissue suggests that this process is directly relevant to understanding signalling in established and native networks. Importantly, examples of mobile vesicle fusion have been very elegantly demonstrated in a variety of developing neuronal systems [21] , [22] , [23] , [24] , [25] , [26] , [27] and this is thought to be an important step in nascent synapse formation [54] . The specific relationship between this immature signalling process and the phenomenon we examine here is not established. Nonetheless, evidence suggests that, at a mechanistic level, these two signalling processes are quite distinct using, for example, different molecular machinery for exocytosis and exhibiting different pharmacological sensitivity [16] . Our ultrastructural data indicates that mobile fusion sites can have characteristics of conventional terminals at the moment of fusion, including closely apposed postsynaptic targets, suggesting that they could have a direct role to play in information transmission. Over the time course of our experiments we did not see evidence to suggest substantial lateral movement of labelled aggregates of postsynaptic markers. This indicates that it is the trafficking of presynaptic vesicles that largely accounts for the apposition of presynaptic markers with postsynaptic proteins observed soon after stimulation. Of course, mobility in terms of single receptors is highly dynamic [55] and we cannot rule out the possibility of coordinated interactions occurring at the level of individual postsynaptic proteins. Importantly, mobile vesicle fusion onto postsynaptic targets would have very different signalling properties compared with conventional terminals. For example, their transmission capabilities should be directly dependent on vesicle traffic: a parameter that appears to be specifically regulated [17] , [56] . Moreover, functional consequences of extrasynaptic signalling might be very different: for example, activating distinct classes or combinations of target receptors compared with conventional terminals—similar to the functional compartmentalization of signalling in chick ciliary ganglia [5] —or perhaps even activate extrasynaptic receptor pools known to contribute to information transmission in hippocampal neurons [57] . This has implications for plasticity [58] or signalling related to disease conditions [59] , [60] . Thus, further knowledge about the mechanisms regulating synaptic vesicle traffic and axonal fusion as well as the specific receptor targets involved in this process will provide new insights into important aspects of neuronal operation. Cell culture and transfections Dissociated hippocampal cultures were prepared from P0-P1 rats by plating neurons on an astrocyte feeder layer, and maintained in BME media with 45% glucose, 2% FCS and B27 supplement. Mature hippocampal neurons were used for experiments after 11–32 days in vitro . Experiments were performed in accordance with the UK-Animal (Scientific Procedures) Act 1986 and complied with local institutional regulations. Neurons were transfected at days in vitro 7–9, using a Ca 2+ phosphate protocol. Unless otherwise stated, all experiments were performed in external bath solution (137 mM NaCl, 5 mM KCl, 2.5 mM CaCl 2 , 1 mM MgCl 2 , 10 mM d-Glucose, 5 mM HEPES, 20 μM 6-cyano-7-nitroquinoxaline-2,3-dione (CNQX), 50 μM d(-)-2-amino-5-phosphonovaleric acid (AP5)) at 25 °C. Labelling and imaging of cultured neurons Recycling synaptic vesicles were labelled using field stimulation (600 APs, 10 Hz) in the presence of the dye (FM1-43 or its fixable analogue FM1-43FX, FM4-64, 10 μM, Molecular Probes). After loading, cells were washed with fresh external bath solution for 10 min to remove surface dye. In some experiments, vesicles were labelled using fluorescently tagged antibodies directed to the vesicle protein synaptoptagmin I (anti-synaptotagmin Oyster550, anti-synaptotagmin CypHer5E, 1:200, Synaptic Systems) using the loading and washing protocol outlined above. Similarly, live labelling of postsynaptic structures (anti-GluR1, Calbiochem; anti-GluR2, Millipore, 1:200; anti-GABA-A receptor β2,3 Chain, Millipore, 1:400) was carried out at 37 °C for 30 min followed by secondary labelling (anti-rabbit or anti-mouse Alexa 488 or 568, 1:100). Plasmid constructs used were ECFP-PSD-95, SypHy2x, SypI-mCherry and GFP-actin. Imaging of living and fixed cells was carried out with an Olympus BX61WI microscope using a X60 1.0 N.A. dipping objective. Excitation and emission filter sets for fluorescent probes were as follows: ECFP-PSD-95, 438/24, 470/22; FM1-43, SypHy2x and GFP-actin, 480/20, 520/35; FM4-64, 470/22, 624/40; SytI-Oyster550, 556/20, 609/54; SypI-mCherry 556/20, 624/40; CypHer5E, 628/40, 692/40. Image analysis was performed using ImageJ ( http://rsb.info.nih.gov/ij/ ) on raw unfiltered images or after filtering (1×1 median filter) applied to the whole image. For each mobile packet, we first characterized the movement dynamics by generating a kymograph from a line profile that traced the axon. The kymograph was then used as a guide to define the region of interest (ROI) for our packet in the time-lapse image sequence. To extract raw fluorescence intensity values for packets, we targeted the packet in the frame before stimulation. An ROI was drawn that encapsulated the packet and flanking axon ( ∼ 1 μm on each side). In the subset of cases where packets continued to move after stimulation, multiple ROIs were used to track fluorescence intensity along the axon, using the kymograph as a guide. Background fluorescence was subtracted from an ROI adjacent to the target packet but that did not include the axon or other structures. For analysis of mobility rates in relation to stimulation, we generated kymographs and overlaid linear profiles that described the lateral movement over time. Movement rates before and after stimulation could be extracted by measuring the angles of the line profile and converting to distance and time units. Quantification of the occurrence of mobile-fusion events relative to dye-loss events at stable synapses was carried out by analysis of kymographs generated from line profiles along discrete axonal segments. Segments ( n =50) were chosen that had a defined stable terminal and a flanking axonal length (3.5 μm) that did not include other stable terminals. Mobile fusion events were only counted if they were mobile before the stimulus and could be distinguished from dye loss at the stable synapse. Curve fitting was carried out with Prism or Igor. Statistical comparisons used appropriate two-tailed t -tests unless otherwise stated. Significance was defined as P <0.05. Acute slice preparation Acute transverse slice preparations of hippocampus (300 μm) were prepared from 18–24 d rats. Presynaptic terminals were labelled using a protocol similar to those described previously [30] , [31] . Briefly, slices were loaded with bath application of FM1-43 (20 μM) in aCSF containing (in mM): 125 NaCl, 2.5 KCl, 25 glucose, 1.25 NaH 2 PO 4 , 26 NaHCO 3 , 1 MgCl 2 , 2 CaCl 2 and 50 μM AP5 (pH 7.3 when bubbled with 95% O2 and 5% CO2). Slices were incubated in FM1-43 solution (3 min) and subsequently a 1,200 AP 10 Hz loading stimulation was delivered using a bipolar tungsten electrode placed near Schaffer collaterals. Two minutes after the end of stimulation slices were washed in continuously perfused aCSF (10 min) and then in the FM-dye chelator ADVASEP-7 (1 mM, Biotium, 1 min). Finally, slices were continuously perfused with aCSF for >20 min. Before FM-dye loading the target CA1 region was chosen on the basis of the electrical response to stimulation recorded with an aCSF-filled glass electrode (2–3 MΩ); to allow postsynaptic responses to be recorded, AMPARs were not blocked in these experiments. Imaging of FM-dye-labelled presynaptic terminals used an Olympus BX51WI microscope equipped with a FV-300 confocal system (Olympus UK), a 488-nm Ar laser and 520/10 emission. Confocal time-lapse image sequences (optical section thickness<1.4 μm) were acquired with 2-second intervals between frames; the rate required to track movements of packets. Immunofluorescence Hippocampal cultures were fixed with either 4% paraformaldehyde in PBS or 4% paraformaldehyde and 1% glutaraldehyde in PBS. The preparations were washed and quenched in 50 mM NH 4 Cl and permeabilized in 0.2% Triton X-100 PBS. After blocking with goat serum, cells were incubated in anti-mouse glutamate (ImmunoStar, 1:2,000) or anti-PSD-95 (Abcam, 1:200), followed by a secondary incubation with goat anti-mouse Alexa 488 or 568 (Invitrogen, 1:500). Coverslips were mounted in fluorescence mounting medium (DAKO) for imaging. Photoconversion and electron microscopy Hippocampal cultures labelled with FM1-43FX were fixed and photoconverted using a previously established protocol [15] , [39] . Briefly, neurons were fixed in 2% PFA/2% glutaraldehyde for 15 min, washed with 100 mM glycine (1 h) followed by NH 4 Cl (1 min) and rinsed in PBS. Photoconversion was obtained by illuminating the samples with 475/40 nm light from a mercury lamp for 12 min in the presence of diaminobenzidine (DAB, 1 mg ml −1 , DAKO). Following photoconversion, samples were osmicated, stained and embedded in EPON (TAAB) [15] , [39] . Embedded samples were sectioned and collected on formvar-coated slot grids. Sections were viewed using a Hitachi-7100 transmission electron microscope and images acquired using a 2,048 × 2,048 CCD camera (Gatan). Micrographs were aligned and reconstructed using Xara Xtreme and Reconstruct (Synapse Web, Kristen M. Harris, http://synapses.clm.utexas.edu/ ). Electrophysiology and calcium imaging Whole-cell recordings were obtained using patch pipettes (3–5 MΩ resistance) filled with 115 mM potassium methylsulphate, 5 mM potassium chloride, 10 mM HEPES buffer, 10 mM creatine phosphate, 2 mM ATP-Mg, 2 mM ATP-Na 2 , 0.3 mM. GTP-Na 2 and 200 μM Oregon Green 488 BAPTA-1 (OGB-1) or Fluo-5F (Molecular Probes). Voltage recordings were carried out using a Multiclamp 700A amplifier and digitized using a Digidata 1320a (Molecular Devices). Electrophysiological traces were visualized and analysed using pClamp software (Molecular Devices). Calcium imaging experiments were carried out using an Olympus BX51WI microscope equipped with a FV-300 confocal system (Olympus UK). SypI-mCherry and OGB-1 or Fluo-5F were excited with a 543 nm HeNe laser and a 488 nm Ar laser (CVI Melles-Groit), respectively. Line scans were obtained at 500–750 Hz using a X60 water immersion objective (1.0 N.A., Olympus UK). The relative changes in fluorescence of OGB-1 or Fluo-5F were quantified as Δ F / F 0 ( t )=( F ( t )− F 0 )/ F 0 , where F 0 is the basal fluorescence calculated averaging the intensity values of 100 ms preceding the action potential for each pixel in the line; %Δ F / F 0 was expressed as a percentage of the fluorescence at the peak of the calcium signal at the synapse. Calcium signals were analysed using Matlab (The Mathworks); peak amplitudes, 10–90% rise and 100% decay times were measured using Igor pro (Wavemetrics) with the Neuromatic package ( www.neuromatic.thinkrandom.com/ ). In experiments to characterize Ca 2+ hotspots and mobile fusion at the same sites, we loaded neurons with the membrane permeable form of OGB-1 (OGB-1-AM, 200 μM, Molecular Probes, 2 h incubation at 37 °C). Synapses were labelled with FM4-64 (600 APs, 10 Hz) as above. Images of OGB-1-AM signal were collected at 50 Hz for 4 s using a CCD system (above) and a single AP was evoked by field stimulation. Time-lapse imaging for FM-dye signal (every 2 s) was initiated immediately after this and the culture destained at 40 Hz. How to cite this article: Ratnayaka, A. et al . Extrasynaptic vesicle recycling in mature hippocampal neurons. Nat. Commun. 2:531 doi: 10.1038/ncomms1534 (2011).